Critical speeding-up in the magnetoelectric response of spin-ice near its monopole liquid–gas transition Competing interactions in the so-called spin-ice compounds stabilize a frustrated ground state with finite zero-point entropy and, interestingly, emergent magnetic monopole excitations. The properties of these monopoles are at the focus of recent research with particular emphasis on their quantum dynamics. It is predicted that each monopole also possesses an electric dipole moment, which allows to investigate their dynamics via the dielectric function ε ( ν ). Here we report on broadband spectroscopic measurements of ε ( ν ) in Dy 2 Ti 2 O 7 down to temperatures of 200 mK with a specific focus on the critical end point present for a magnetic field along the crystallographic [111] direction. Clear critical signatures are revealed in the dielectric response when, similarly as in the liquid–gas transition, the density of monopoles changes in a critical manner. The dielectric relaxation time τ exhibits a critical speeding-up with a significant enhancement of 1/ τ as the temperature is lowered towards the critical temperature. Besides demonstrating the magnetoelectric character of the emergent monopole excitations, our results corroborate the unique critical dynamics near the monopole condensation transition. The magnetic rare earth ions of the spin-ice compounds such as Dy 2 Ti 2 O 7 form a lattice of corner-sharing tetrahedra. The strong influence of crystal fields forces the magnetic moments to point along the axis connecting the centres of adjacent tetrahedra giving rise to a description in terms of effective Ising spins. In zero magnetic field, the ground state is characterized by a two-in/two-out spin state configuration, that is, there are two spins for each tetrahedron that point inwards and two that point outwards. The ground state, however, is not unique as there is a multitude of possible realizations of this two-in/two-out arrangement giving rise to a finite zero-point entropy. Given the resemblance to the proton configurations of water–ice, this peculiar magnetism is known as spin-ice [1] , [2] , [3] . Flipping a single spin breaks the two-in/two-out ice rule for two adjacent tetrahedra: the resulting magnetic dipole excitation decomposes into an emergent magnetic monopole and antimonopole pair that interacts via a long-range magnetic Coulomb law [4] , [5] . Spin-ice thus offers a rare example of fractionalized excitations in a three-dimensional (3D) material. Recently, it has been pointed out by Khomskii [6] that each magnetic monopole is also accompanied by an electric dipole. The presence of a magnetic monopole on a tetrahedron results in an electric dipole moment either because of a spontaneous charge redistribution or because of a magnetoelastic coupling. This dipole moment always points along the corner of the tetrahedron that is occupied by the spin, which is singled out by the one-in/three-out or the one-out/three-in configuration, see Fig. 1a,b . Single spin–flip processes amounting to a hop of a single monopole from one tetrahedron to another as well as multiple spin–flip processes that only redistribute the one-in/three-out or one-out/three-in configurations on a tetrahedron are accompanied by a change of the net electric dipole moment. The dynamics of the electric dipoles on magnetic monopoles thus leads to characteristic fluctuations of the electric polarization that, in principle, can be investigated with the help of the dielectric function ε ( ν ). First experimental indications for a magnetoelectric coupling in Dy 2 Ti 2 O 7 were reported by Saito et al. [7] However, in their work the permittivity was only measured for a fixed frequency of 1 kHz. In the present work, we use broadband dielectric spectroscopy and present measurements of ε ( ν ) in Dy 2 Ti 2 O 7 for a wide range of frequencies, 1 Hz< ν <1 MHz, and temperatures down to 200 mK. 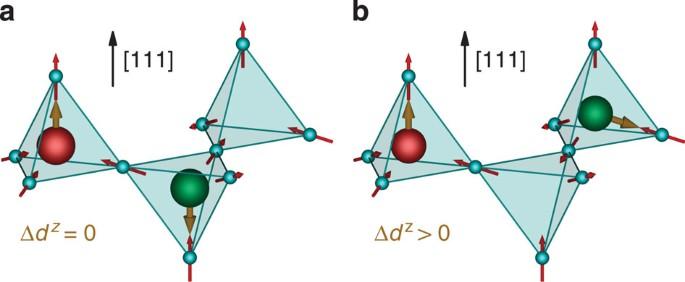Figure 1: Electric dipoles on magnetic monopoles. (a) Corner-sharing network of tedrahedra in spin-ice with an Ising spin (red arrow) located on each corner. Breaking of the ice rules results in an effective magnetic monopole/antimonopole pair (red and green balls) each of which carries an electric dipole moment (brown arrow). (b) The hopping of a monopole corresponds to flipping a single Ising spin, here giving rise to a non-vanishing net electric dipole moment Δdz. Figure 1: Electric dipoles on magnetic monopoles. ( a ) Corner-sharing network of tedrahedra in spin-ice with an Ising spin (red arrow) located on each corner. Breaking of the ice rules results in an effective magnetic monopole/antimonopole pair (red and green balls) each of which carries an electric dipole moment (brown arrow). ( b ) The hopping of a monopole corresponds to flipping a single Ising spin, here giving rise to a non-vanishing net electric dipole moment Δ d z . Full size image Magnetic and dielectric response A comparison between the magnetic and dielectric response in Dy 2 Ti 2 O 7 is shown in Fig. 2a,b . The spin dynamics up to kHz frequencies was already intensively explored by magnetic a.c.-susceptibility χ ( ν ) measurements [8] , [9] , [10] , [11] , [12] , [13] . In zero magnetic field the corresponding spin relaxation time is found to be temperature-independent between 3 and 12 K but increases exponentially at lower temperatures as the ice rules start to establish themselves. A spectrum of χ ( ν ) is shown in the upper frame of Fig. 2a . The loss peak in the imaginary part χ ′′( ν ) at a temperature of 2 K is located at , and the resulting relaxation time, τ =1/(2 πν p ), is in nice agreement with previously reported results [9] , [10] , [11] , [12] , [13] . Although our spectral range for χ ( ν ) is also experimentally limited to ν ≤1 kHz, it is already apparent that the real part χ ′( ν ) levels off at a finite value at higher frequencies. One expects that a second relaxation process, which has not been detected yet, eventually leads to a vanishing of χ ′( ν ) at even larger ν . The first, slow relaxation process has been associated with the Brownian diffusion of monopole excitations [5] , [12] . 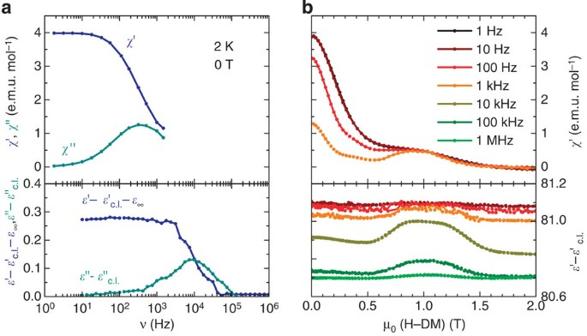Figure 2: Magnetic and dielectric response. (a) Spectra of the complex magnetic a.c.-susceptibilityχ(ν) (upper frame) and of the complex permittivityε(ν) (lower frame) at 2 K in zero magnetic field. The dielectric function was corrected for a constant lossεc.l.(ν) and a background contributionε∞as described in the text. (b) The real parts of magnetic a.c.-susceptibility (upper frame) and permittivity (lower frame) as a function of internal magnetic field,Hi=H−DM, along the [111] axis atT=2 K measured for frequencies between 1 Hz and 1 MHz. Figure 2: Magnetic and dielectric response. ( a ) Spectra of the complex magnetic a.c.-susceptibility χ ( ν ) (upper frame) and of the complex permittivity ε ( ν ) (lower frame) at 2 K in zero magnetic field. The dielectric function was corrected for a constant loss ε c.l. ( ν ) and a background contribution ε ∞ as described in the text. ( b ) The real parts of magnetic a.c.-susceptibility (upper frame) and permittivity (lower frame) as a function of internal magnetic field, H i = H − DM , along the [111] axis at T =2 K measured for frequencies between 1 Hz and 1 MHz. Full size image A spectrum of the dielectric response ε ( ν ) is shown in the lower frame of Fig. 2a . We find that ε ( ν ) is insensitive to the slow relaxation process that governs χ ( ν ). Instead, its relaxation dynamics is roughly two orders of magnitude faster with a loss peak in ε ′′( ν ) located at roughly . At this point, it is however unclear whether this relaxation process is related to magnetism or rather has a non-magnetic origin. Monopole liquid–gas transition In order to identify the magnetic contribution to the dielectric response, we investigated its magnetic field dependence. Particularly interesting is the application of a magnetic field along the [111] direction. For intermediate values, a quarter of all spins then align with the magnetic field at low temperatures because of the Zeeman energy. The remaining spins occupy sites of decoupled two-dimensional (2D) Kagome lattices. The ground-state manifold consistent with the ice rules is still degenerate and thus realizes Kagome ice . At a critical internal field of μ 0 H i,c =1 T in Dy 2 Ti 2 O 7 (refs 14 , 15 , 16 , 17 ), it becomes advantageous to break the ice rules and to quench the remaining zero-point entropy in order to minimize the Zeeman energy further. Correspondingly, at the transition monopoles proliferate and are accommodated into the magnetic ground state at larger fields. Neglecting the magnetic Coulomb force among monopoles, this transition is approximated by a 2D Ising model in a longitudinal field [18] . However, the long-range interaction promotes quantum fluctuations so that the transition becomes first-order and also extends to finite T (ref. 4 ). The resulting line of first-order transitions terminates at a critical end point at a finite temperature T c =360 mK (refs 14 , 15 , 16 , 17 ). It was argued in ref. 19 that the universality of this end point is equivalent to the one in critical uniaxial ferroelectrics that show mean-field behaviour with logarithmic corrections. In Kagome-ice, the low-energy monopole excitations carry an electric dipole that is parallel or antiparallel aligned with the applied magnetic field, see Fig. 1a . Other configurations such as in Fig. 1b have an excitation energy of ~4 K close to the critical field so that they are frozen out at lower temperatures. On the other hand, in the limit of large fields each tetrahedron houses a monopole whose electric dipoles are antiferroelectrically ordered with respect to each Kagome plane. Correspondingly, it was suggested in ref. 6 that antiferroelectricity is a secondary-order parameter of the transition at H i,c with the concomitant signatures in ε ( ν ). Field and temperature dependence of relaxation processes The magnetic field dependence of the magnetic response χ ′( ν ) at T =2 K is shown in the upper frame of Fig. 2b for frequencies up to 1 kHz. At small fields χ ′( ν ) is strongly dispersive but it becomes practically frequency-independent at higher fields. This change of dispersion is less attributed to a field dependence of the relaxation rate but rather to a quench of the slow relaxation process as the magnetic field increases towards H i,c , that is, the weight of the loss peak in χ ′′( ν ) is suppressed with increasing H i [11] , [12] . The field dependence of the dielectric response to an a.c. electric field longitudinal to the [111] axis is displayed in the lower frame of Fig. 2b . Again, ε ( ν ) is insensitive to the slow relaxation dominating χ ( ν ) but only exhibits faster relaxation that becomes visible for frequencies exceeding 1 kHz. At the same time, a pronounced magnetic field dependence appears with a maximum close to the critical field. Full spectra of the dielectric response are presented in Fig. 3 for selected magnetic fields and temperatures in complete agreement with previously reported results [7] . The spectra contain a constant field-independent contribution to ε ′′, which translates via the Kramers–Kronig relations to giving rise to a constant negative slope in the permittivity on a logarithmic frequency scale, see Supplementary Note 1 . Such a constant loss is known from other titanate-based quantum-paraelectric materials such as SrTiO 3 (ref. 20 ). It has been attributed to quantum tunnelling between narrow off-centred positions of the Ti ions, which are also responsible for the very high absolute value of the low-temperature permittivity of about ε ∞ ≈80. A comparison of the dielectric loss with measurements on the non-magnetic iso-structural compound Y 2 Ti 2 O 7 at 600 mK plotted in grey in Fig. 3b shows that the peak is absent while a constant loss contribution remains. The detailed results on Y 2 Ti 2 O 7 are shown in Supplementary Fig. 1 . This constant loss was subtracted from the data shown in Fig. 2 . 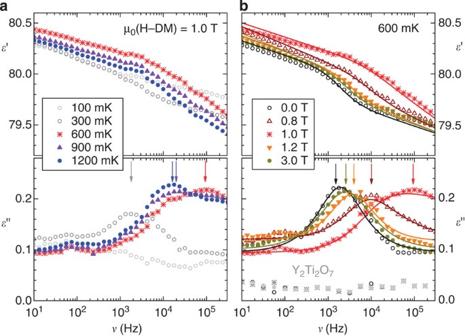Figure 3: Full spectra of the dielectric response in Dy2Ti2O7. (a) Selected temperatures close to the critical field and (b) selected internal magnetic fieldsHiatT=600 mK. The step-like features in the real partε′ and the corresponding loss peaks in the imaginary partε′′ shift withTandHi. A maximal peak frequencyνp≈100 kHz is obtained in the immediate vicinity of the critical end point. The solid lines inbare fits to the Havriliak–Negami relaxation function21together with a background and constant loss contributions as described in the text. Figure 3: Full spectra of the dielectric response in Dy 2 Ti 2 O 7 . ( a ) Selected temperatures close to the critical field and ( b ) selected internal magnetic fields H i at T =600 mK. The step-like features in the real part ε ′ and the corresponding loss peaks in the imaginary part ε ′′ shift with T and H i . A maximal peak frequency ν p ≈100 kHz is obtained in the immediate vicinity of the critical end point. The solid lines in b are fits to the Havriliak–Negami relaxation function [21] together with a background and constant loss contributions as described in the text. Full size image After considering the large constant background and the constant loss, the remaining dielectric relaxation was modelled using a Havriliak–Negami function, which in principle can be related to an asymmetrically broadened distribution of relaxation times (see ref. 21 and Supplementary Note 2 ). It yields a very good description of the complex permittivity spectra as demonstrated in Fig. 3b . The full set of fitting parameters is also given in Supplementary Fig. 2 . The most important parameter characterizing the relaxational dynamics is the position, ν p , of the loss peak (see arrows in Fig. 3 ) that defines a dielectric relaxation rate 1/ τ =2 πν p . The dependences of ν p ( T , H i ) for temperatures, T , below 2 K and internal magnetic fields, μ 0 H i , up to 2 T is shown in Fig. 4 . Away from the critical field, μ 0 H i,c =1 T, the relaxation rate depends only weakly on the magnetic field, see Fig. 5a and Supplementary Fig. 3 for a detailed discussion. However, a strong magnetic influence indisputably appears close to the critical field. The relaxation rate changes dramatically as a function of field and temperature and it reflects the critical behaviour associated with the monopole liquid–gas end point. We therefore conclude that the dielectric dynamics is sensitive to the criticality of magnetic monopoles close to their condensation transition. 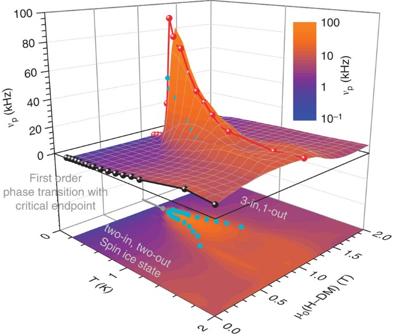Figure 4: Peak frequency of the dielectric loss spectra. νp=1/(2πτ) as a function of temperature,T, and internal fieldHi=H−DMalong the [111] axis. The critical end point temperature isTc=360 mK. The black and red curve markνp(T) at zero and critical field; the blue dots mark the positions of full-width at half-maximum (FWHM) of theνp(Hi) curves at different temperatures. Figure 4: Peak frequency of the dielectric loss spectra. ν p =1/(2 πτ ) as a function of temperature, T , and internal field H i = H − DM along the [111] axis. The critical end point temperature is T c =360 mK. The black and red curve mark ν p ( T ) at zero and critical field; the blue dots mark the positions of full-width at half-maximum (FWHM) of the ν p ( H i ) curves at different temperatures. 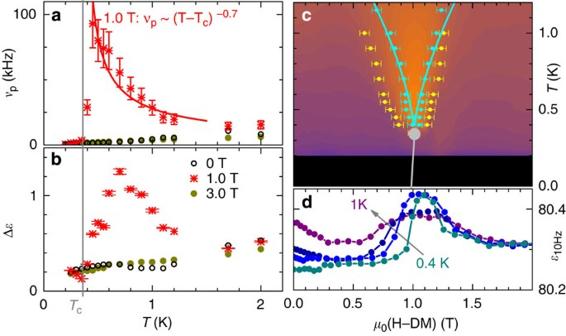Figure 5: Signatures of criticality. (a) Temperature dependence of the relaxation frequencyνpand (b) of the relaxation strength Δεat three different internal magnetic fields. (c) (Hi,T) diagram and contour plot of the peak frequencyνp=1/(2πτ) of the dielectric loss (same colour legend as inFig. 4). The position of FWHM ofνp(Hi) (blue dots) approximately obeyT~Tc~|Hi−Hi,c|2/3scaling (blue line). (d) Quasistatic permittivityε10Hzmeasured atν=10 Hz. The inflection points of its field dependence are marked in (c) as yellow dots. The origin of error bars is discussed in detail inSupplementary Fig. 4. Full size image Figure 5: Signatures of criticality. ( a ) Temperature dependence of the relaxation frequency ν p and ( b ) of the relaxation strength Δ ε at three different internal magnetic fields. ( c ) ( H i , T ) diagram and contour plot of the peak frequency ν p =1/(2 πτ ) of the dielectric loss (same colour legend as in Fig. 4 ). The position of FWHM of ν p ( H i ) (blue dots) approximately obey T ~ T c ~| H i − H i,c | 2/3 scaling (blue line). ( d ) Quasistatic permittivity ε 10Hz measured at ν =10 Hz. The inflection points of its field dependence are marked in ( c ) as yellow dots. The origin of error bars is discussed in detail in Supplementary Fig. 4 . Full size image Besides establishing the magnetoelectric coupling in spin-ice, the results of Fig. 4 also reveal unexpected critical dynamics. Away from the critical field, the relaxation rate decreases monotonically with temperature, see Supplementary Fig. 3 for more details. However, as the critical end point is approached, the relaxation changes dramatically with a sharp increase in ν p . This implies that the polarization decorrelates faster close to criticality. Assuming critical dynamic scaling, we can relate the relaxation time to the correlation length, τ ~ ξ z , via the dynamical exponent z . At the critical field the correlation length is assumed to diverge as a function of temperature, with the correlation length exponent ν ξ >0, so that Usually, the dynamical exponent z is positive resulting in the canonical behaviour of critical slowing-down. Here we find instead a negative dynamical exponent implying a critical speeding-up of the dynamics. Close to the critical temperature, this speeding-up is particularly dramatic as a function of field with ν p ( H i ) growing by two orders of magnitude. From a fit within the temperature range from 450 mK to 1.2 K we can estimate the exponents to be approximately ν ξ z ≈−0.7, see Fig. 5a . The critical speeding-up close to the critical end point in spin-ice might be a generic property of monopole dynamics that is not only reflected in the dielectric but might be also detectable in the magnetic response. In fact, recent results for the dynamical susceptibility by Takatsu et al. [13] obtained down to 0.5 K provide first evidence that the relaxation of the magnetization also exhibits a pronounced speeding-up. The corresponding inverse relaxation time 1/ τ at low T was found to increase sharply as a function of magnetic field, similarly as our results for ν p in Fig. 4 . Close to the critical end point, the relaxation peak in χ ′′ even shifts to frequencies beyond 1 kHz so that a detailed analysis of the critical dynamics of the magnetization and, in particular, of its temperature dependence could not be performed yet. For a direct comparison with our results for the dynamical exponent z presented in Fig. 5a measurements of χ ( ν ) for much larger frequencies are therefore necessary. Nevertheless, for the limited frequency range considered in ref. 13 , it was argued that single spin–flip Monte Carlo dynamics already accounts for the speeding-up, hinting at a critical enhancement of monopole diffusion. We continue with a discussion of the crossover scales associated with the positions of the full-width at half-maximum of the function ν p ( H i ), which yield the blue dots in Fig. 4 . These crossover lines first follow the mean-field prediction for the primary order parameter [19] , T − T c ~| H i − H i,c | 2/3 , as shown by the blue solid lines in Fig. 5c . A similar scaling close to the end point is also observed in the specific heat [15] . Closer inspection, however, reveals deviations very close to the critical temperature. Indeed, critical speeding-up comes to a halt at a temperature of 450 mK just before T c =360 mK, and ν p ( T ) abruptly drops towards zero, see Fig. 5a This sudden qualitative change of behaviour could have different origins. It might be attributed either to inhomogeneous demagnetization fields smearing the critical behaviour or a slight misalignment of the applied field with respect to the [111] axis. Alternatively, it could indicate a crossover to a more conventional behaviour of critical slowing-down. The relaxation process is also very asymmetric with respect to the critical temperature. It is indistinguishable from the non-critical background for T < T c . The weight of the dielectric loss, that is, the relaxation strength Δ ε is shown in Fig. 5b . Again, the weight at zero field and 3 T are barely distinguishable but a strong enhancement appears close to the critical field. As a function of decreasing temperature, the weight starts to increase at ~1.5 K but peaks at ~700 mK before dropping back to the non-critical background. The location of this peak position emphasizes the qualitative change of the relaxation dynamics upon approaching the critical temperature as already observed in the relaxation rate. The quasistatic limit of the dielectric response, ε 10 Hz , measured at ν =10 Hz is shown in Fig. 5d . As pointed out in ref. 7 , the two plateaus emerging at low temperatures can be related to a magnetic renormalization of the permittivity, δε (0)~‹ M 2 › and reflect the constant magnetization of Kagome ice and its saturation at low and high fields, respectively. The peak of ε 10 Hz close to the critical field gives rise to inflection points whose positions are marked as yellow dots in Fig. 5c . Interestingly, the resulting crossover appears to be markedly different from the one extracted from the full-width at half-maximum of ν p ; however, it is reminiscent of the one observed in the adiabatic susceptibility in ref. 12 , see Supplementary Fig. 5 and the Supplementary Discussion for further information. The emergent magnetic monopoles in spin-ice are accompanied by an electric dipole moment giving rise to intrinsic magnetoelectric coupling [6] . We confirmed this magnetoelectricity in Dy 2 Ti 2 O 7 and, in addition, demonstrated that the dielectric dynamics gets dramatically modified close to the monopole liquid–gas transition resulting in a critical speeding-up. In order to confirm its precise link to monopoles, detailed measurements of the critical magnetic dynamics at frequencies extending 1 kHz are now called for [13] . Besides elucidating a peculiar aspect of the dynamical critical behaviour of monopole condensation, our findings provide a proof of principle for dielectric spectroscopy of monopoles in spin-ice. Sample preparation Single crystals of Dy 2 Ti 2 O 7 were grown using a floating zone method. The structural characterization by X-ray diffraction revealed phase purity and the expected cubic structure. The samples were prepared as thin platelets normal to the [111] direction with a typical thickness of d ≈0.35 mm and an area of A ≈10 mm 2 . Magnetic and dielectric measurements The measurements of the complex dielectric permittivity were performed in the frequency range from 1 Hz to 1 MHz, employing a frequency–response analyzer Novocontrol A LPHA -A with stimuli of typically 1 V mm −1 . For these measurements, contacts of silver paste were applied at opposite sides of the crystal platelets. The samples were oriented with magnetic and electric fields in the crystalline [111] direction. The magnetic field range up to 3.5 T and the temperature range from 100 mK to 5 K for the dielectric measurements were covered using a QuantumDesign PPMS magnetocryostat and an Oxford Kelvinox 3 He/ 4 He dilution refrigerator. The magnetic a.c.-susceptibility measurements were performed in a QuantumDesign MPMS SQUID with a.c.-Option with a.c.-magnetic field stimuli of two Oe parallel to the applied d.c.-field along [111] direction. Demagnetization correction For technical reasons, dielectric measurements were performed on a disc-like sample of Dy 2 Ti 2 O 7 with a very high demagnetization factor D resulting in substantial demagnetization fields within the sample. Therefore, the internal magnetic field strength H − DM has been calculated numerically using magnetization data for Dy 2 Ti 2 O 7 in [111] magnetic field published in ref. 17 , the radia software package provided by the ESRF [22] , and the dimensions of the rectangular sample. How to cite this article: Grams, C. P. et al. Critical speeding-up in the magnetoelectric response of spin-ice near its monopole liquid–gas transition. Nat. Commun. 5:4853 doi: 10.1038/ncomms5853 (2014).